Rebalancing of internally generated carriers for mid-infrared interband cascade lasers with very low power consumption The interband cascade laser differs from any other class of semiconductor laser, conventional or cascaded, in that most of the carriers producing population inversion are generated internally, at semimetallic interfaces within each stage of the active region. Here we present simulations demonstrating that all previous interband cascade laser performance has suffered from a significant imbalance of electron and hole densities in the active wells. We further confirm experimentally that correcting this imbalance with relatively heavy n -type doping in the electron injectors substantially reduces the threshold current and power densities relative to all earlier devices. At room temperature, the redesigned devices require nearly two orders of magnitude less input power to operate in continuous-wave mode than the quantum cascade laser. The interband cascade laser is consequently the most attractive option for gas sensing and other spectroscopic applications requiring low output power and minimum heat dissipation at wavelengths extending from 3 μm to beyond 6 μm. Many ubiquitous commercial technologies such as telecommunications and optical disc drives rely on mature near-infrared and visible diode lasers as key components. On the other hand, it is widely viewed as inevitable that mid-infrared (which we define here as λ =3–6 μm) semiconductor lasers must suffer from excessive threshold current densities as a consequence of their high non-radiative recombination rates. However, the impact of the rapid non-radiative decay is commonly overestimated, in part because the threshold carrier density needed to achieve gain is significantly lower in a narrow-gap material owing to its smaller density of states. Although the photon loss also tends to be higher at longer wavelengths, it can be offset by the gain from cascaded multiple quantum wells (QWs), each fed by the same current in a series arrangement. This reduces the threshold power density in comparison with conventional diodes with multiple QWs connected in parallel, by lowering the voltage drop over the series resistance. The cascading mechanism was popularized by the well-known quantum cascade laser (QCL) [1] , [2] , [3] , [4] , [5] , which in fact has a very short (picosecond, ps) upper lasing level lifetime characteristic of intersubband transitions. In spite of this liability and thanks in part to the exceptionally weak temperature dependence of its threshold, QCLs now realize multi-watt CW output powers from single narrow ridges operating at room temperature (RT) [2] , [6] . Nevertheless, the most significant observable consequence of the short carrier lifetime is that the lowest pulsed threshold power density reported at RT has been P th ≈12 kW cm −2 (refs 6 , 7 ) This value has not improved in over three years, even as other QCL performance characteristics have advanced significantly. Mid-infrared interband cascade lasers (ICLs) [8] , [9] generally have the advantage of much longer lifetimes characteristic of the interband active transition [10] , although with considerably stronger temperature dependence. For many important applications such as battery-operated fielded systems that require relatively low output powers and are operated very close to the lasing threshold, the threshold power density at RT represents one of the most important figure of merit. However, a full evaluation of the potential of the ICL has not been possible thus far because an inadequate understanding of the ICL's internal physics always resulted in suboptimal device performance. In what follows we present the first complete theoretical description of the ICL's unique internal carrier generation and transport processes, which are critical to its high-temperature operation. We then show that by implementing a new design that features a complete rebalancing of the electron and hole densities in the active QWs, laboratory devices exhibiting P th as low as 0.35 kW cm −2 at RT have been demonstrated. We further point out that the reconfigured ICL approach may similarly benefit other types of semiconductor lasers with QW active regions. Conventional and cascaded lasers The carrier-generation mechanism of the ICL differs significantly from those operative in conventional diode lasers and QCLs. 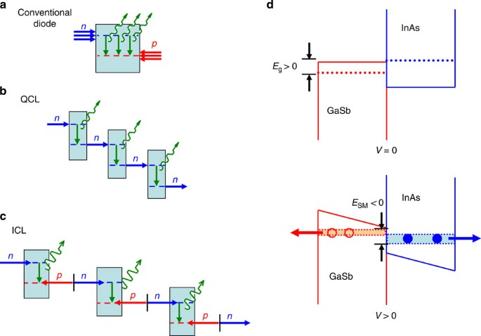Figure 1: Schematic diagrams of the carrier injection processes. Electron injection is indicated with blue arrows, and hole injection with red arrows. Photon emission is indicated with green arrows. Blue (red) dashed lines stand for subbands in the conduction (valence) bands. The diagrams are shown for: (a) a conventional diode laser, where the multiple arrows stand for potential injection into multiple QWs, (b) a QCL and (c) an ICL, where the black vertical lines indicated the location of the SMIF within each stage. The energy alignment for adjacent InAs and GaSb QWs in equilibrium and under bias is shown in (d), where the solid blue and red lines are the conduction and valence-band edges, respectively, in bulk materials. In the absence of a bias, quantum confinement leads to an energy gapEgbetween the lowest conduction and highest VB states (blue and red dotted lines, respectively), whereas under bias a semimetallic overlapESMis imposed that leads to the generation of equal electron and hole densities, represented by the solid blue and open red circles, respectively. The applied field also causes both carrier types to flow away from the interface (arrows), requiring that they be replaced on an ongoing basis to maintain quasi-thermal equilibrium populations. In a conventional diode illustrated in Figure 1a , electrons are injected into the conduction band (CB) from one contact and holes are injected into the valence band (VB) at the opposite contact, and the injected current divides between the multiple active QWs. The minimum threshold voltage ( V th ) scales with the photon energy as ħω / q , where q is the electron charge. The active region is typically undoped, although modulation doping has been introduced in some cases to lower the threshold current density or to improve high-speed operation [11] , [12] , [13] , [14] , [15] , [16] , [17] . Figure 1: Schematic diagrams of the carrier injection processes. Electron injection is indicated with blue arrows, and hole injection with red arrows. Photon emission is indicated with green arrows. Blue (red) dashed lines stand for subbands in the conduction (valence) bands. The diagrams are shown for: ( a ) a conventional diode laser, where the multiple arrows stand for potential injection into multiple QWs, ( b ) a QCL and ( c ) an ICL, where the black vertical lines indicated the location of the SMIF within each stage. The energy alignment for adjacent InAs and GaSb QWs in equilibrium and under bias is shown in ( d ), where the solid blue and red lines are the conduction and valence-band edges, respectively, in bulk materials. In the absence of a bias, quantum confinement leads to an energy gap E g between the lowest conduction and highest VB states (blue and red dotted lines, respectively), whereas under bias a semimetallic overlap E SM is imposed that leads to the generation of equal electron and hole densities, represented by the solid blue and open red circles, respectively. The applied field also causes both carrier types to flow away from the interface (arrows), requiring that they be replaced on an ongoing basis to maintain quasi-thermal equilibrium populations. Full size image In the QCL illustrated in Figure 1b , the current flow is entirely due to electrons and passes through each active QW. This reduces the threshold current density ( J th ) at the expense of a higher threshold voltage that must exceed Mħω / q , where M (>1) is the number of stages. Cascading reduces the threshold power density as long as there is a series resistance (or a non-ohmic voltage drop) [18] , and J th does not suffer appreciably from the introduction of the cascaded geometry. The cascading in a QCL also provides preferential injection into the upper lasing subband and fast extraction from the lower lasing subband [19] . Although the electrons populating the upper lasing subband of each stage come primarily from the injector doping in the preceding stage, the internal electric field resulting from the charge separation remains modest because the threshold carrier density is <10 10 cm −2 rather than ~10 12 cm −2 as in an interband QW laser at RT. Although the carrier density is approximately two orders of magnitude lower, the upper lasing level lifetime is over three orders of magnitude shorter (<1 ps versus >1 ns), which results in much higher threshold current densities in the QCL. ICL design In contrast to the conventional diode and QCL, the ICL generates both electrons and holes internally, at an interface with energy alignment that varies from semiconducting to semimetallic with applied bias V ( Fig. 1c ). It is the only known laser with this feature. The internal generation is facilitated by the alignment of the CB minimum in InAs at an energy ~0.2 eV below the VB maximum of GaSb [20] . As depicted in Figure 1d , the applied electric field leads to a transition from a positive energy gap induced by quantum confinement back to the semimetallic alignment with band overlap E SM ( V ) that allows both electron states in the InAs QW and hole states in the GaSb QW to be populated in thermal quasi-equilibrium. The external electric field sweeps the generated carriers away from the junction, with holes flowing to the left and electrons to the right. To replenish the carriers removed by the field, thereby maintaining quasi-equilibrium, equal numbers of additional electrons and holes must be regenerated continuously at the semimetallic interface (SMIF). In the ideal design, the separation between the quasi-Fermi levels (QFLs) in successive stages (equal to the single-stage voltage drop) must simultaneously produce an optical gain that compensates the photon loss in the cavity ( E Fi − E Fi+1 ≥ ħω ≥ E g , with the electron QFL in stage i , E Fi , being equal to the hole QFL in stage i −1) and internally generate a quasi-equilibrium carrier density n int = p int ≈ E SM m r */ πħ 2 (ref. 18 ), where m r * is the reduced density-of-states mass. When added to any carriers produced by extrinsic doping, the resulting electron and hole densities produce the QFL separation specified above. Although the first condition is a property of the active QWs, the second one follows from the design and doping of the (multiple) electron and hole QWs on both sides of the SMIF. This voltage-balancing condition, which requires careful design optimization, has never been considered or treated explicitly in the prior ICL literature. Excessive voltage drops or free-carrier absorption losses due to carrier accumulation can develop if the design deviates appreciably from this equality in either direction. 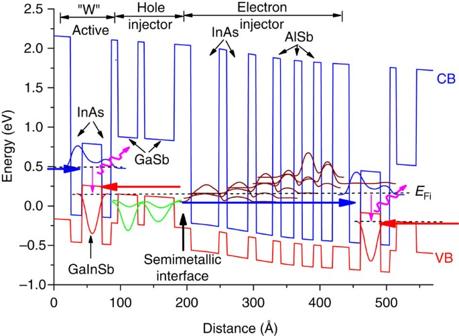Figure 2: Illustrative band diagrams of the complete ICL active core. Band diagram for 1½ stages of the ICL structure considered in this work. Probability densities and zone-center energies (indicated by the wavefunction zero points) for some of the most important subbands are superimposed. The probability densities for the active electron (hole) subbands are indicated with blue (red) lines, while those for the injector-electron (hole) subbands are indicated with wine-coloured (green) lines. The blue (red) arrows indicate the direction of the electron (hole) motion in the structure. The dashed lines indicate the position of the quasi-Fermi levels in each stage. The layer structure of one period starting with the barrier separating the electron injector and the active region is as follows: 25 Å AlSb/17 Å InAs/30 Å Ga0.65In0.35Sb/14 Å InAs/10 Å AlSb/30 Å GaSb/10 Å AlSb/45 Å GaSb/25 Å AlSb/42 Å InAs/12 Å AlSb/32 Å InAs/12 Å AlSb/25 Å InAs/12 Å AlSb/20 Å InAs/12 Å AlSb/17 Å InAs/12 Å AlSb/17 Å InAs. The identity of the various layers, key parts of the structure and the position of the SMIF are also indicated. Figure 2 shows that these multiple QWs are comprised of the chirped InAs/AlSb electron injector and two active InAs electron QWs [21] of the next stage on one side of the SMIF (green arrow) and the GaSb/AlSb hole injector and the active GaInSb hole QW on the other. Both sets of QWs must be designed for consistency with the voltage-balancing condition, which differs considerably from design considerations for the QCL. A second role of the hole injector is to present a barrier to direct electron current flow that bypasses the VB [18] , [22] . Our analysis assumes that carrier thermalization on both sides of the SMIF is much faster than the carrier lifetime. Although the previous reports did not treat the extent to which internally generated carriers transfer to the active QWs upon thermalization, the critical nature of this phenomenon is revealed by our analysis. Figure 2: Illustrative band diagrams of the complete ICL active core. Band diagram for 1½ stages of the ICL structure considered in this work. Probability densities and zone-center energies (indicated by the wavefunction zero points) for some of the most important subbands are superimposed. The probability densities for the active electron (hole) subbands are indicated with blue (red) lines, while those for the injector-electron (hole) subbands are indicated with wine-coloured (green) lines. The blue (red) arrows indicate the direction of the electron (hole) motion in the structure. The dashed lines indicate the position of the quasi-Fermi levels in each stage. The layer structure of one period starting with the barrier separating the electron injector and the active region is as follows: 25 Å AlSb/17 Å InAs/30 Å Ga 0.65 In 0.35 Sb/14 Å InAs/10 Å AlSb/30 Å GaSb/10 Å AlSb/45 Å GaSb/25 Å AlSb/42 Å InAs/12 Å AlSb/32 Å InAs/12 Å AlSb/25 Å InAs/12 Å AlSb/20 Å InAs/12 Å AlSb/17 Å InAs/12 Å AlSb/17 Å InAs. The identity of the various layers, key parts of the structure and the position of the SMIF are also indicated. Full size image One way to satisfy the voltage-balancing condition is to align the ground states of the electron and hole injectors with those of the active QWs. However, in that case, most of the internally generated electrons and holes reside in quasi-equilibrium in the respective injectors rather than in the active QWs, in part because of the opposing internal field. Empirically, we have found that alignment with the active QWs is required only for the electron injector. The holes generated at the SMIF can transfer efficiently to the active GaInSb hole QW so long as the injector QW states lie no more than 100 meV (≈4 k B T ) below the active hole subband energy. Therefore, in quasi-equilibrium, the hole population residing in the GaSb injector QW states is negligible. Rebalancing the electron and hole densities Although most previous ICL designs introduced moderate n -doping into the electron injector [23] , the rationale seemed questionable, as the internally generated carrier densities significantly exceeded the doping densities. 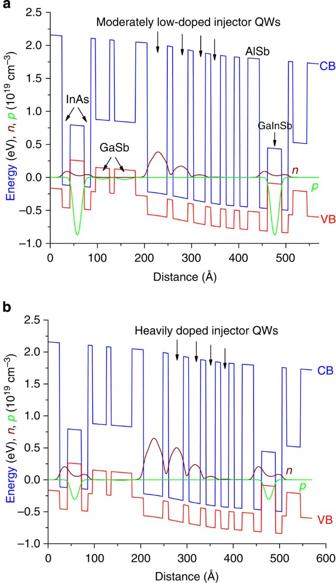Figure 3: Calculated quasi-equilibrium carrier density distributions. The electron (wine-coloured) and hole (green) density distributions are shown for: (a) a conventional ICL design with four InAs electron injector QWs doped moderately with Si to 4×1017cm−3, and (b) a rebalanced design in which four injector QWs are doped much more heavily to 5×1018cm−3. The blue and red lines indicate the conduction- and valence-band bulk band edges, respectively. Positions of the doped QWs in each structure are indicated by the arrows. In the typical example of Figure 3a , our self-consistent quasi-equilibrium distribution calculations found that because the injected electrons tend to reside mostly in the injector, whereas nearly all of the injected holes transfer to the active GaInSb QW, the active hole population substantially outnumbers that for electrons. A priori this large hole/electron density ratio is neither advantageous nor disadvantageous, as the impact on threshold current density depends on the relative recombination coefficients for ppn versus nnp Auger processes, and to a lesser extent on the relative electron and hole free-carrier absorption cross-sections. As such a scenario is advantageous only in the event that hole processes are far weaker than the corresponding electron processes, we should explore the alternative option of rebalancing the electron and hole densities. Figure 3: Calculated quasi-equilibrium carrier density distributions. The electron (wine-coloured) and hole (green) density distributions are shown for: ( a ) a conventional ICL design with four InAs electron injector QWs doped moderately with Si to 4×10 17 cm −3 , and ( b ) a rebalanced design in which four injector QWs are doped much more heavily to 5×10 18 cm −3 . The blue and red lines indicate the conduction- and valence-band bulk band edges, respectively. Positions of the doped QWs in each structure are indicated by the arrows. Full size image This can be accomplished by n -doping the electron injector QWs much more heavily. In Figure 3b , the doping is strategically shifted towards the active region to maximize the electron transfer, and its level is increased by over an order of magnitude to 5×10 18 cm −3 . The figure indicates that this radical increase rebalances the quasi-equilibrium electron and hole populations in the active QWs so that their densities are comparable. Such a distribution will be advantageous whenever multi-hole Auger processes contribute appreciably to the total Auger rate. Pulsed characterization of broad-area lasers To test the hypothesis that heavy intentional doping of the injector QWs may substantially lower the lasing threshold by rebalancing the active electron and hole concentrations, we grew a series of five-stage ICL wafers, emitting at λ =3.6–3.9 μm, to designs incorporating this new feature (Methods). Table 1 compiles calculated and measured properties of these structures for pulsed operation at T =300 K. We find that all six of the devices with heavily doped injector QWs (samples 4–9) exhibited much lower threshold current densities, and also lower internal losses deduced from the slope efficiencies above threshold, than any of the first three “conventional” devices with injectors doped at a more moderate level. For example, the threshold current density decreased from J th ~400 A cm −2 (equivalent to the best ever reported before the present study) to as low as 167 A cm −2 . Not shown in Table 1 is that the threshold voltage also decreased, from V th ~2.5 V for the conventional structures to ~2.1 V (the ideal lower limit is Mħω / q ~1.6–1.7 V). Characteristic temperatures of T 0 ~43 K and T 1 ~121 K were typical for these devices in the 300–350 K range. Table 1 Experimental and theoretical characteristics of the samples with varying injector doping levels. Full size table Following the successful demonstration that all of the heavily doped devices listed in Table 1 exhibited much lower threshold currents and voltages (the injector-region doping level was the only major difference between them), samples redesigned to impose carrier rebalancing at other emission wavelengths were also grown. 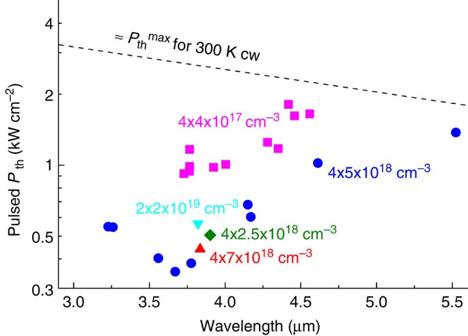Figure 4: Pulsed threshold power density versus wavelength for five-stage ICLs. All the measurements were performed at a temperature of 300 K. The doping is as follows: four wells doped to 4×1017cm−3(magenta squares), four wells doped to 2.5×1018cm−3(olive diamond), four wells doped to 5×1018cm−3(blue circles), four wells doped to 7×1018cm−3(red triangle) and two wells doped to 2×1019cm−3(cyan inverted triangle). The wavelength was varied by changing the InAs layer thickness in the active region and in parts of the electron injector, while keeping the rest of the structure fixed. All devices used the same standard broad-area geometry with 150 μm ridge width and 2 mm cavity length. The theoretical estimate of maximum threshold power density for which RT CW operation should be possible once narrow ridges are processed (dashed curve) was derived assuming a thermal impedance-area product of 4 K cm2kW−1and parameterizing the temperature dependence of the threshold power density as an exponential curve at various wavelengths. Figure 4 illustrates pulsed threshold power densities P th = J th V th for broad-area ICLs at T =300 K as a function of wavelength. The structures with rebalanced carrier densities are seen to substantially outperform the earlier ICLs at all λ , with P th remaining below the estimated power density required for RT CW operation (dashed curve) out to λ =5.5 μm. Thus far, the lowest threshold power densities (≈0.35 kW cm −2 ) have been observed for the λ =3.6–3.9-μm devices listed in Table 1 . Figure 4: Pulsed threshold power density versus wavelength for five-stage ICLs. All the measurements were performed at a temperature of 300 K. The doping is as follows: four wells doped to 4×10 17 cm −3 (magenta squares), four wells doped to 2.5×10 18 cm −3 (olive diamond), four wells doped to 5×10 18 cm −3 (blue circles), four wells doped to 7×10 18 cm −3 (red triangle) and two wells doped to 2×10 19 cm −3 (cyan inverted triangle). The wavelength was varied by changing the InAs layer thickness in the active region and in parts of the electron injector, while keeping the rest of the structure fixed. All devices used the same standard broad-area geometry with 150 μm ridge width and 2 mm cavity length. The theoretical estimate of maximum threshold power density for which RT CW operation should be possible once narrow ridges are processed (dashed curve) was derived assuming a thermal impedance-area product of 4 K cm 2 kW −1 and parameterizing the temperature dependence of the threshold power density as an exponential curve at various wavelengths. Full size image CW characterization of narrow-ridge lasers The improved pulsed performance implied that ICLs with rebalanced carrier densities should exhibit enhanced CW operation as well. Selecting Wafer 6 from Table 1 for narrow-ridge processing (Methods), ridges were fabricated with nominal widths of 5, 8 and 11 μm, cavity lengths of 0.5 or 4 mm and a high-reflection (HR) coating on the back facet. Output facets were either anti-reflection (AR) coated or uncoated (U). 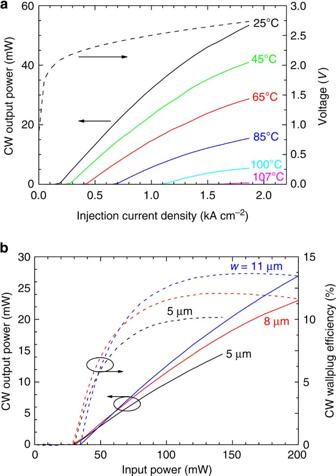Figure 5: Measured light–current–voltage characteristics for narrow-ridge ICLs. (a) CW light-current curves at heat-sink temperatures of 25, 45, 65, 85, 100 and 107 °C (solid lines from top to bottom) and the current–voltage curve at 25 °C (dashed) for a narrow-ridge ICL with 8-μm ridge width, 4 mm cavity length, and one HR-coated and one uncoated facet. The emission wavelength changed from 3.68–3.88 μm from the lowest to the highest operating temperature. (b) CW output power (solid) and wallplug efficiency (dashed) at a heat-sink temperature of 25 °C versus input electrical power for narrow ridges of three widths (the curves for 11 μm are shown with blue lines, 8 μm red and 5 μm black) and a cavity length of 0.5 mm with one uncoated facet and one HR-coated facet. In panelblasing is obtained for input powers as low as 29 mW. Figure 5a shows CW L–I characteristics for an 8 μm×4 mm ridge with HR/U facets at a series of temperatures (as well as the I – V characteristic at T =25 °C). Note that CW operation is maintained at 107 °C, which is by far the highest T max cw ever reported for an interband semiconductor laser emitting beyond 3 μm. The emission wavelength at that temperature is λ =3.88 μm. An 11 μm×4 mm device with HR/AR coatings generated a CW output power of 158 mW, which is nearly a factor of 3 higher than any previous ICL result at RT. Figure 5b indicates that when the cavity length was shortened to 0.5 mm (with HR/U facets), the wall-plug efficiency at 25 °C reached 13.5%. The same short cavities achieved CW lasing at a remarkably low-input power of 29 mW. Two devices with each ridge width were tested, and found to provide quite similar performance characteristics. Figure 5: Measured light–current–voltage characteristics for narrow-ridge ICLs. ( a ) CW light-current curves at heat-sink temperatures of 25, 45, 65, 85, 100 and 107 °C (solid lines from top to bottom) and the current–voltage curve at 25 °C (dashed) for a narrow-ridge ICL with 8-μm ridge width, 4 mm cavity length, and one HR-coated and one uncoated facet. The emission wavelength changed from 3.68–3.88 μm from the lowest to the highest operating temperature. ( b ) CW output power (solid) and wallplug efficiency (dashed) at a heat-sink temperature of 25 °C versus input electrical power for narrow ridges of three widths (the curves for 11 μm are shown with blue lines, 8 μm red and 5 μm black) and a cavity length of 0.5 mm with one uncoated facet and one HR-coated facet. In panel b lasing is obtained for input powers as low as 29 mW. Full size image Theoretical analysis Our simulations can be applied to the experimental results discussed above using the Auger recombination coefficients for multielectron and multihole processes and the internal loss as fitting parameters. 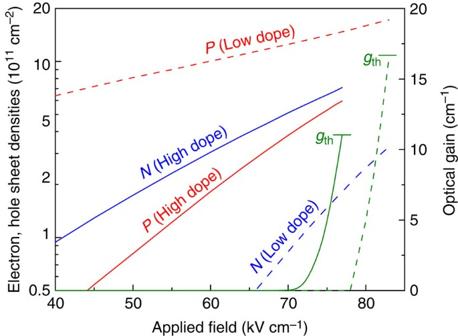Figure 6: Calculated modal optical gain and carrier densities. Modal optical gain (given by the product of the material gain and the optical confinement factor, olive lines) plotted on the right axis and the electron (blue) and hole (red) sheet densities plotted on the left axis in one stage of the ICL structure as a function of applied electric field for devices with four InAs electron injector QWs doped moderately with Si to 4×1017cm−3(dashed lines) and a rebalanced design in which four injector QWs are doped much more heavily to 5×1018cm−3(solid lines). The curves are terminated at the threshold point (corresponding to the experimental loss and the fitted Auger coefficient) of each structure. The calculations were performed for lattice and carrier temperatures of 300 K. Figure 6 compares the resulting electron and hole densities in the active QWs versus applied electric field for the conventional moderately doped structure (4×10 17 cm −3 ) as well as the heavily doped (5×10 18 cm −3 ) design that rebalances the carrier populations. In the former case, far more holes than electrons are present at all applied fields, as in quasi-equilibrium most electrons populate the electron injector rather than the active QWs as discussed above. On the other hand, rebalancing via heavy n -doping tips the hole/electron population ratio to a value less than unity. Considerably higher gain is then generated at all applied fields (green curves). The calculations also confirm that the voltage drop per stage in an ideal rebalanced ICL may exceed the photon energy by as little as ≈12 meV. This small excess is required to overcome the internal loss plus the mirror loss of 4.5 cm −1 for a 2-mm-long cavity with uncoated facets. On the other hand, QCLs require voltage margins of many k B T (100–150 meV) to prevent backfilling of the lower lasing subband [24] . Figure 6: Calculated modal optical gain and carrier densities. Modal optical gain (given by the product of the material gain and the optical confinement factor, olive lines) plotted on the right axis and the electron (blue) and hole (red) sheet densities plotted on the left axis in one stage of the ICL structure as a function of applied electric field for devices with four InAs electron injector QWs doped moderately with Si to 4×10 17 cm −3 (dashed lines) and a rebalanced design in which four injector QWs are doped much more heavily to 5×10 18 cm −3 (solid lines). The curves are terminated at the threshold point (corresponding to the experimental loss and the fitted Auger coefficient) of each structure. The calculations were performed for lattice and carrier temperatures of 300 K. Full size image We noted above that a large hole/electron population ratio is preferable when Auger recombination is strongly dominated by nnp processes. However, the data summarized in Table 1 indicate that the lowest thresholds are obtained when the active electron and hole concentrations are roughly equal. This finding provides the first experimental confirmation that ppn and nnp Auger processes have similar strengths in type-II active regions, which is consistent with the available theoretical evidence [25] . For the samples in Table 1 with the heaviest doping levels, the threshold electron density is much higher than the threshold hole density ( n th >> p th ). As in the opposite scenario of prior art ICLs without rebalancing ( p th >> n th ), the lack of available states in one of the bands requires a large (exponential) increase in the number of states in the other band if the same optical gain is to be maintained. As a result, J th has a minimum at intermediate doping levels, for which n th and p th are of the same order of magnitude. However, the optimum point does not necessarily correspond to n th = p th because of the larger density of states in the VB and secondary differences in the free-carrier absorption cross-sections and Auger coefficients. Fitting the data in the Table 1 to a simple model (Methods) gives that the nnp contribution to the net Auger coefficient is γ 3 nnp /γ 3 = γ 3 nnp /( γ 3 ppn + γ 3 nnp )=0.51. The net Auger coefficients derived from the current density threshold for each device, listed in the final column of Table 1 , fall in the narrow range γ 3 =2.8–3.4×10 −27 cm 6 s −1 . The dependence of this value on hole/electron concentration ratio is negligible, as γ 3 ppn and γ 3 nnp are equal to within experimental uncertainty. However, the fitting nevertheless finds that a slightly higher electron density is preferred. The trend of the losses extracted from slope efficiencies for the various samples implies that the free-carrier absorption cross-section is smaller for electrons than for holes. The high threshold current densities of longer wavelength semiconductor lasers have long been viewed as unavoidable, as a small energy gap is accompanied by much stronger non-radiative recombination and much higher free-carrier absorption loss. Nevertheless, the J th values as low as 170 A cm −2 demonstrated in this work fall within the typical range for near-infrared diodes. The material properties that enable this result are a lower threshold carrier density (associated with a smaller density of states) and suppressed Auger recombination relative to bulk materials with similar gaps. In spite of these considerations, the optimal performance levels can be realized only in the cascaded geometry and in conjunction with rebalancing to optimize the hole/electron density ratio. The maximum CW operating temperature of 107 °C achieved by one of the rebalanced narrow ridges is 35 °C higher than the best previous result for NRL ICLs, and 87 °C beyond any T max cw reported for all other ICLs or other interband semiconductor laser emitting beyond 3.4 μm. Furthermore, the wallplug efficiency of 13.5% at RT has been exceeded by QCLs only recently, and thus far only by two research groups (Northwestern [2] and Pranalytica) in spite of the intense activity being devoted to QCLs. The minimum input power of 29 mW shown in Figure 5b is far lower than any QCL value reported to date. The best QCL result of 830 mW was demonstrated using a partially transmissive HR coating [26] . This approach has not yet been applied to ICLs and can potentially lower their input powers as well, although the output power will also scale down. The more common QCL values of 2–5 W are two orders of magnitude larger than the results now attainable for ICLs. Also advantageous is the ICL's much lower bias requirement of <2.5 V, which compares with 10–15 V for most QCLs. This is because the reported ICLs use only five stages, whereas QCLs need 30–40 stages to reach J th low enough for RT CW operation. A major implication of the significant input-power suppression is that battery lifetimes for fielded sensing systems can be extended by approximately two orders of magnitude. Packaging and other design constraints also relax considerably when the operating power budget is reduced. As long as there is no requirement for high-output power, this advantage applies to any wavelength at which ambient-temperature operation is attainable. Our preliminary wavelength study ( Fig. 3 ) indicates that it may include the entire λ =3–6 μm spectral range. Use of the rebalancing scheme described here has enabled room-temperature CW operation of the ICL at λ =5.7 μm, to be reported elsewhere. Powers of ~1 mW are generally adequate for chemical sensing so that the devices can be assumed to operate very close to threshold. Although the input power is very important for battery-operated systems, a narrow spectral linewidth is also required for most spectroscopic applications. The short non-radiative lifetime that dominates the threshold of the QCL also appears to have the beneficial effect of significantly reducing the spectral width [27] , [28] . Although distributed-feedback lasers processed from ICL wafers using earlier-generation designs have produced 29 mW or more of single-mode CW output at thermoelectric cooler temperatures [29] , the true spectral linewidth of the distributed-feedback ICLs has not been measured to date, although spectrometer-resolution-limited lines have been observed [29] . We finally note that the rebalancing scheme proposed above may be applied to any semiconductor laser that relies on internal generation to produce electrons and holes. This may encompass, for example, antimonide emitters with type-I active QWs (such as InGaAsSb/Al(GaAs)Sb) in addition to the InAs/GaInSb type-II structures of the present work. SMIFs are also readily available in the HgCdTe and lead-salt systems, and even the energy gap for InGaAs/GaAsSb QWs lattice matched to InP may be sufficiently narrow to enable near-IR ICLs, for example, at telecom wavelengths. At this point, QCLs remain preferable for mid-infrared applications requiring high CW output powers at wavelengths beyond about 4 μm. However, we anticipate that the performance characteristics reported above for the new generation of carrier-rebalanced ICLs will position these devices as the lasers of choice for those mid-infrared applications in which compactness, low cost and low-power budget are paramount. Simulation The electron and hole densities and the gain were obtained from a self-consistent simulation of the CB and VB structure at a given applied field in conjunction with Poisson's equation. The zone-center subband energies and wavefunctions were calculated using a two-band k·p method with electron and light-hole states included and a separate one-band method for heavy holes. The tabulated in-plane dispersion relations for typical electron and hole QWs were used to speed up the simulation. The optical gain for a given field was obtained from the Fermi carrier statistics used in the self-consistent solver and the optical matrix elements calculated from the wavefunctions using the standard formalism [30] . The Auger coefficients were obtained from a fit to the experimental threshold current densities and slope efficiencies (using an internal efficiency of η i =76% determined from a cavity-length study [10] , with minor changes in η i having almost no impact on the main results) to the following functional form: η i J th = q ( γ 3 ppn p th 2 n th + γ 3 nnp n th 2 p th ). Here n th and p th are the threshold electron and hole densities, respectively, obtained by dividing the threshold sheet densities needed to achieve a modal gain equal to the photon losses in the cavity by the normalization thickness of 100 Å. First the total Auger coefficient γ 3 = γ 3 ppn + γ 3 nnp and the ratio r n = γ 3 nnp /γ 3 were fit for all the samples in Table 1 . Then the Auger coefficients for the individual samples were estimated from the threshold current densities using the expression above and a fixed value of r n determined from the original fit. Please note that the Auger coefficients derived in some of our previous works [10] , [22] were too low because of an erroneous overestimate of the threshold carrier concentrations. Device Fabrication ICL wafers were grown on n -GaSb (100) substrates in a Riber Compact 21T MBE System using previously described methods [31] . The five-stage active region was enclosed by two 500-nm-thick n -GaSb separate-confinement layers (SCLs), whereas the top and bottom n -doped cladding layers were 24.3 Å InAs/23 Å AlSb superlattices. Transition regions were introduced between the substrate and the bottom cladding, the claddings and the SCLs, the SCLs and the active core, and the top cladding and the top contact, to smooth out abrupt shifts of the CB offset. Contact lithography and wet chemical etching were used to produce 150-μm-wide ridges for pulsed characterization. The etch proceeded to the GaSb SCL below the active region and used a mask with intentional lateral corrugation of the ridge sidewalls to frustrate the parasitic lasing modes [32] . Narrow ridges with varying widths were fabricated by photolithography and reactive-ion etching using a Cl-based inductively coupled plasma process that stopped within the bottom GaSb SCL region. The ridges were subsequently cleaned with a phosphoric-acid-based wet etch to minimize the damage from the dry etch. A 200-nm-thick Si 3 N 4 layer was deposited by plasma-enhanced chemical vapour deposition, and a top-contact window etched back using SF 6 -based inductively coupled plasma. Next, 100 nm of SiO 2 was sputtered to block occasional pinholes in the Si 3 N 4 . The ridges were metallized and then electroplated with 5 μm of Au. Various cavity lengths were cleaved, and facet coatings were applied to some devices. The HR coating comprised of 46-nm-thick Al 2 O 3 and 100-nm-thick Au layers. The AR coating comprised of a 524-nm-thick Al 2 O 3 ( λ /4) layer. Device Characterization The devices were mounted epitaxial side up on a copper heat sink attached to a thermoelectric cooler. The devices were characterized in CW mode or pulsed using a repetition rate of 3 kHz and pulse width of 200 ns. Several devices from each wafer were tested to validate that the reported thresholds are representative of a particular wafer. For devices from a given wafer, the reproducibility of threshold current densities was typically within 5%. How to cite this article: Vurgaftman I. et al . Rebalancing of internally generated carriers for mid-infrared interband cascade lasers with very-low-power consumption. Nat. Commun. 2:585 doi: 10.1038/ncomms1595 (2011).